Social heuristics shape intuitive cooperation Cooperation is central to human societies. Yet relatively little is known about the cognitive underpinnings of cooperative decision making. Does cooperation require deliberate self-restraint? Or is spontaneous prosociality reined in by calculating self-interest? Here we present a theory of why (and for whom) intuition favors cooperation: cooperation is typically advantageous in everyday life, leading to the formation of generalized cooperative intuitions. Deliberation, by contrast, adjusts behaviour towards the optimum for a given situation. Thus, in one-shot anonymous interactions where selfishness is optimal, intuitive responses tend to be more cooperative than deliberative responses. We test this ‘social heuristics hypothesis’ by aggregating across every cooperation experiment using time pressure that we conducted over a 2-year period (15 studies and 6,910 decisions), as well as performing a novel time pressure experiment. Doing so demonstrates a positive average effect of time pressure on cooperation. We also find substantial variation in this effect, and show that this variation is partly explained by previous experience with one-shot lab experiments. Cooperation, where individuals pay costs to benefit others, has been a major topic of interest in the natural and social sciences for the last half century. Cooperation in non-zero-sum contexts increases social welfare but is costly to the cooperator. Thus, a tension exists between individual and collective interests, creating a social dilemma. Much work has tried to explain why evolution would favour cooperation [1] , [2] , [3] , [4] , [5] , and under what circumstances modern humans are more or less likely to cooperate [6] , [7] , [8] , [9] , [10] . More recently, scholars have begun to examine the cognitive processes that support or undermine cooperation: How does the choice to cooperate (or not) actually get made? One approach considers cooperative decision making from within a dual-process cognitive framework [11] , [12] , which conceptualizes decisions as resulting from the interaction between more intuitive versus reflective processes [13] , [14] , [15] , [16] . Intuitive processes are typically characterized as being fast, automatic, effortless and emotional. Reflective processes, by contrast, are typically slower and more controlled, effortful and deliberative. Applying this dual-process framework to cooperation presents the following question about the cognitive basis of prosociality: When confronted with a social dilemma, is our more automatic response to be selfish, such that we cooperate through deliberative self-control? Or are we predisposed towards cooperation, with reflection leading to self-interest and more selfish choices? Or alternatively, is there no internal conflict between intuition and reflection in the context of cooperation? These questions have been left unresolved by seemingly contradictory previous findings: some studies show a positive effect of time pressure on cooperation [12] while others show no effect [17] . Thus, a theory is needed that can predict when intuition will, and will not, have an effect on cooperation. We propose such a theory of the connection between intuition and cooperation, the social heuristics hypothesis (SHH), and in doing so reconcile these previous results. The SHH builds on previous research demonstrating cultural differences in cooperative behaviour [8] , [18] , [19] , [20] , [21] . Likewise, the SHH builds on theories according to which social norms are internalized in the form of automatic behavioural dispositions [22] , [23] , [24] , [25] . The SHH integrates these ideas with dual-process theories that contrast intuitive heuristic processes with more deliberative processes [13] , [14] , [15] , [16] , [26] , [27] . According to the SHH, people internalize strategies that are typically advantageous and successful in their daily social interactions. They then bring these automatic, intuitive responses with them into atypical social situations, such as most laboratory experiments. More reflective, deliberative processes may then override these generalized automatic responses, causing subjects to shift their behaviour towards the behaviour that is most advantageous in context. Thus, the SHH can be thought of as taking theories related to social emotions and norm internalization [22] , [23] , [24] and making them explicitly dual process: instead of valuing options based on a single utility function (with emotional inputs), the SHH contends that people often have two competing sets of preferences, one more intuitive and the other more reflective. Furthermore, the SHH emphasizes the role of generalization from personal experience, thus connecting individual-level learning to individual-level behaviour [28] , [29] . How, then, does this SHH perspective apply to cooperation? In one-shot anonymous settings, such as most typical lab experiments, there is no financial incentive to cooperate. Thus, according to the SHH, reflection should favour selfishness here. The contexts where our intuitions developed, however, were (and are) rarely one-shot and anonymous: instead, daily life typically involves factors such as repetition, reputation and the threat of sanctions, all of which can make cooperation in one’s long term self-interest [9] . In places where these factors, together with institutional rules that support interactions with strangers, make cooperation advantageous, individuals develop intuitions that favour such cooperation. Because most economic experiments are conducted with populations drawn from such places [8] , one-shot anonymous interactions in the lab can elicit cognitive conflict: intuitive responses ‘spill over’ from typical situations (and often favour cooperation), whereas competing reflective responses favour selfishness. Thus, the SHH predicts that on average, intuition will favour cooperation. Based on the SHH, however, we would not expect this conflict to occur for all people. For example, subjects whose intuitions were shaped in contexts where cooperation is not supported will internalize defection as their default response. Thus for these subjects, no cognitive conflict exists: both intuition and reflection favour selfishness, and cooperation should be relatively low regardless of whether subjects decide intuitively or reflectively. These could be people who, for example, developed under social norms that allow or promote selfishness, or corrupt institutions where free-riding is incentivized [8] , [20] , [21] . A similar logic applies to people who live in cooperative environments, but have substantial previous experience with the ‘atypical’ lab setting. These individuals will have had the opportunity to develop new automatic responses tailored to these alternative settings and, unlike naïve subjects, will not rely on the intuitions from daily experiences. For such subjects, no cognitive conflict should exist as they have already developed new intuitions specifically suited to the problem at hand. Put differently, the SHH posits that intuitive cooperation results from the overgeneralization of intuitive heuristics developed in daily life, and greater experience with lab experiments allows subjects to readjust their intuitions to the laboratory setting. In sum, the SHH therefore predicts that intuition will promote cooperation among some people (and some groups), and will have no effect on other people (and other groups): intuition is predicted to favour cooperation among those who (i) are from daily life environments that favour cooperation, and (ii) have little prior experience with laboratory experiments. But based on the SHH, intuition should never decrease average cooperation relative to reflection in one-shot anonymous social dilemmas. To evaluate these predictions, we analyse a large corpus of data applying time constraints to economic cooperation games. These data were generated by our group over a 2-year period. Time constraints provide a method, widely used in experimental psychology, for inducing subjects to rely more on intuition (through time pressure) or reflection (through time delay) [30] , [31] , [32] , [33] , [34] . This is because a key property of intuitive, heuristic processing is that it is automatic and operates relatively quickly. Controlled, deliberative processing, by contrast, is typically slower, in some cases because competing automatic responses must be overridden. Forcing people to decide quickly reduces their ability to reflect and gives them less opportunity to override their intuitive responses. Conversely, forcing people to stop and think has the opposite effect, allowing for more deliberation. Of course, the application of time pressure does not result in purely intuitive responding; nor does the enforcement of a delay result in purely reflective responding. Reflection may fail to override deeply held intuitions, and some subjects may engage in substantial reflection even under time pressure. Rather, by comparing time pressure and time delay we can reveal the dominant directions of the effects of intuitive versus reflective processing. Our aggregate analysis examines data from all 15 time constraint studies conducted by our group between February 2011 and February 2013, starting with the two studies reported in Rand Greene Nowak (2012) (ref. 12 ) (hereafter RGN; the first two such experiments we ran); 6,913 decisions by 5,831 unique individuals in total. While each of these studies varies in its details, they all involve the application of time pressure/delay to cooperation decisions. (Most of these experiments involve a Public Goods Game (PGG) where subjects choose how much money to contribute to a common pool, with contributions doubled and split equally among the subject and three other group members.) By aggregating across them all, we can perform a strong test of the predictions of the SHH: both the positive effect of time pressure on cooperation on average, as well as the predicted study to study variation in that effect (sometimes positive, sometimes null, but never negative). We then complement our aggregate analysis with an additional PGG experiment that explicitly examines a potential moderating factor suggested by the SHH and the results of our aggregate analysis: previous experience with economic game experiments. Aggregate level analysis We begin by evaluating the SHH’s prediction that promoting intuition via time pressure should increase cooperation on average. To do so, we examine aggregate behaviour over all 15 studies. 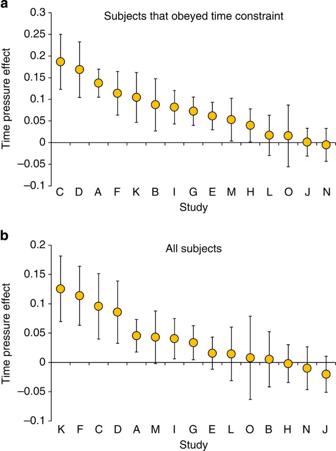Figure 1: The effect of time pressure on cooperation varies from large and positive to null but is never negative. The effect of time pressure on cooperation is disaggregated by study: shown is mean (normalized) cooperation level in the time pressure condition minus mean cooperation level in the time delay condition for each study, sorted in decreasing order. For studies that crossed time pressure with a second manipulation, we pool across secondary manipulations. (a) Only including subjects that obeyed the time constraint and therefore were successfully treated. (b) Including all subjects. Error bars represent robust s.e.m. clustered on subject, taken from a time pressure dummy in a linear regression run for each study. Number of observations by study: A=680, B=163, C=315, D=211, E=801, F=48, G=751, H=601, I=548, J=666, K=210, L=296, M=196, N=603, O=163. SeeTable 6for further details of each study. Regressions restricting to subjects who obeyed the time constraint (and therefore whose cognitive processing was successfully manipulated, as in RGN) are shown in Table 1 . Considering the average frequency of cooperation aggregated across all studies, we find a significant positive effect of time pressure, either without controls for demographics, comprehension and round (column 1: linear regression with robust standard error (s.e.) values; coefficient=0.069, P <0.0001; this translates into a 21.5% increase in contribution over time delay when normalizing at the study level by average time delay contribution) or with these controls (column 2: linear regression with robust standard errors; coefficient=0.069, P <0.0001). We continue to find this significant time pressure effect when excluding the two studies previously published in RGN (columns 3 and 4), or when excluding studies that used games other than the PGG (columns 5 and 6). 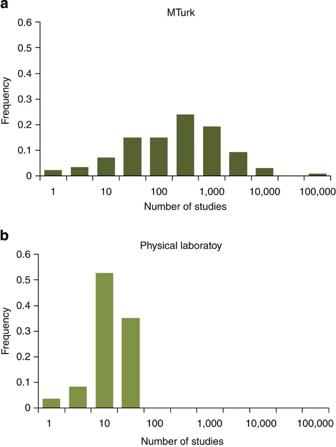Figure 2: Subjects on MTurk are vastly more experienced than subjects in conventional physical laboratories. Shown is the distribution of self-reported total number of studies completed by a sample of 291 MTurk subjects (a) and 118 subjects from the Harvard Decision Sciences Laboratory subject pool (b). Table 2 shows that a qualitatively equivalent significant positive effect of time pressure on cooperation when including the 20% of decisions where subjects did not obey the time constraint (that is, took too long under time pressure, or responded too quickly under time delay). This robustness is important for demonstrating causality [17] . We also note that our results are robust to excluding subjects who did not answer all comprehension questions correctly (linear regression with robust s.e. values; obeyed time constraint: P <0.0001 with or without controls; all subjects: P =0.002 with or without controls), indicating that confusion is not driving the time pressure effect we observe. Table 1 Regression results for cooperation as a function of time pressure focusing on subjects that obeyed the time constraint. Full size table Table 2 Regression results for cooperation as a function of time pressure including all subjects. Full size table Thus we confirm the prediction of the SHH that, on average, time pressure increases cooperation, demonstrating a causal link between intuitive processing and cooperative choice. We also consistently find that (i) subjects who fail the comprehension questions cooperate more, (ii) older subjects cooperate more, (iii) subjects from India cooperate less (17% less of the endowment spent on cooperating on average compared with subjects residing in the United States), and (iv) cooperation decreases with round number in the one experiment that involved multiple rounds of random re-matching (round=1 for all decisions in all other studies). Variation across studies in time pressure effect We now turn from the average effect of time pressure to evaluate the SHH’s prediction about study-level variation in that effect: across studies, the effect of time pressure is predicted to vary from strongly positive to no significant effect, but not to be significantly negative in any studies. To assess this prediction, Fig. 1 shows the effect size (mean difference in cooperation between time pressure and time delay groups) for each study. We see that some studies find a large positive effect of time pressure on cooperation, some find smaller positive effects of time pressure and still others find no significant effect. But none of the 15 studies conducted finds a significant negative effect of time pressure on cooperation. Examining Fig. 1a shows that six studies find a significant positive effect of time pressure, P <0.05; two studies find a marginally significant positive effect, P <0.1; six studies find a non-significant positive effect, P >0.1; and only one study (study N) finds a negative effect, which is extremely small and far from significant: coefficient=−0.005, P =0.89 ( P -values generated using linear regression with robust s.e. values). Regarding effect sizes, nine studies reveal an increase in cooperation of more than 10% under time pressure, relative to time delay. Thus, the data presented in Fig. 1 confirm the predictions of the SHH regarding variation in effect size. Figure 1: The effect of time pressure on cooperation varies from large and positive to null but is never negative. The effect of time pressure on cooperation is disaggregated by study: shown is mean (normalized) cooperation level in the time pressure condition minus mean cooperation level in the time delay condition for each study, sorted in decreasing order. For studies that crossed time pressure with a second manipulation, we pool across secondary manipulations. ( a ) Only including subjects that obeyed the time constraint and therefore were successfully treated. ( b ) Including all subjects. Error bars represent robust s.e.m. clustered on subject, taken from a time pressure dummy in a linear regression run for each study. Number of observations by study: A=680, B=163, C=315, D=211, E=801, F=48, G=751, H=601, I=548, J=666, K=210, L=296, M=196, N=603, O=163. See Table 6 for further details of each study. Full size image The variation across studies shown in Fig. 1 raises the question of what factors determine whether time pressure increases cooperation. In other words, what are the moderators of the time pressure effect? Here we provide evidence for one moderator predicted by the SHH: level of prior experience with one-shot anonymous economic games. The SHH posits that intuitive cooperation is the result of overgeneralization: strategies that are advantageous in typical situations involve repetition, reputation and sanctions spill over into atypical one-shot anonymous interactions. By this logic, substantial prior experience with one-shot lab games will allow subjects to remodel their default behaviour in these games, undermining the intuitive cooperation effect. Amazon mechanical Turk subjects have become highly experienced As a preliminary to our examination of experience as a potential moderator of cooperative behaviour, we explore the effect of changes in the overall level of experience of the subject pool. Of our 15 studies, 12 were conducted using the online labour market Amazon Mechanical Turk (MTurk) [35] , [36] , [37] , [38] , [39] , [40] (reconstructing Fig. 1 using only the studies run on MTurk gives qualitatively similar results). One of the two original RGN experiments was run on MTurk, in February 2011. At that time, the use of MTurk for academic studies was relatively rare: most of the methods papers popularizing MTurk did not appear until later in 2011 or 2012 (refs 35 , 36 , 37 , 38 , 39 ). Over the 2 years following the initial RGN experiment, the use of MTurk amongst social scientists has become extremely common. As a result of this popularization, there is a reason to believe that the MTurk subject pool has become highly experienced with academic studies. To assess this conjecture quantitatively, in April 2013, we surveyed 291 MTurk workers, asking them to report the number of studies in which they had participated. We restricted to subjects residing in the United States and, following a common quality control practice on MTurk, to participants with a minimum 75% approval rating for their prior MTurk work. For comparison with the traditional physical lab, we also administered the same questions to 118 subjects from the Harvard Decision Sciences Laboratory subject pool. The results are shown in Fig. 2 . Figure 2: Subjects on MTurk are vastly more experienced than subjects in conventional physical laboratories. Shown is the distribution of self-reported total number of studies completed by a sample of 291 MTurk subjects ( a ) and 118 subjects from the Harvard Decision Sciences Laboratory subject pool ( b ). Full size image The median MTurk worker reported participating in 300 academic studies in total, 20 of which occurred in the past week (importantly, this figure includes only academic studies—the median number of total MTurk jobs of any kind was 1500). In contrast, the median physical lab subject reported participating in 15 academic studies in total, only 1 of which occurred in the past week. Thus the MTurk subject pool is vastly more experienced than our offline subject pool, with the median MTurker completing more studies in a single week than the median lab subject has ever completed (Rank-sum, P <0.0001 for both total studies and studies in the last week). A qualitatively similar pattern is seen when asking specifically about participation in studies where subjects can affect the earnings of others (as a proxy for economic game experience): the median MTurk subject participated in 10 such studies, 1 of which occurred in the past week, whereas the median lab subject participated in 4 such studies, none of which occurred in the past week (Rank-sum, P <0.0001 for both total studies and studies in the last week). Thus, the MTurk subject pool has been transformed from naïve to highly experienced over the time period spanned by our 15 studies. This may have led to at least two different changes that could undermine the time pressure effect originally observed in RGN. First, it is more likely that subjects will already be familiar with our specific experimental paradigm. This is particularly true after the publication of RGN, as our exact instructions are included in the Supplementary Methods and have been adopted by numerous groups doing research on MTurk. Second, an increasing prevalence of economic game experiments (as well as many other types of psychology experiments) makes it likely that subjects will be familiar more generally with experimental paradigms in which conflicts exist between intuitive and reflective processes. Thus subjects will have had an opportunity to adjust their default responses to fit these games, reducing the conflict between automatic and deliberative decisions. Finally, it is also possible that time pressure is less able to prevent experienced individuals from deliberating: having done many such experiments before, they may be able to effectively reflect within the 10-s window allowed under time pressure (and may be more resistant to other manipulations aimed at reducing reflection). An increasingly experienced subject pool reduces cooperation under time pressure Given that MTurk subjects have become increasingly experienced with academic studies, the SHH predicts that cooperation under time pressure will have systemically decreased over the 2-year period spanned by our studies, as intuitive cooperation was undermined. Conversely, cooperation under time delay is predicted to remain constant, as reflection leads to selfishness in both naïve and experienced subjects. To evaluate this prediction, we perform a regression predicting cooperation in the 12 MTurk studies, and examine the interaction between time pressure and the date on which the subject made his or her decision (measured in days and normalized to 0 on the first day of the RGN experiment). Specifically, we predict a negative interaction between time pressure and date: among time pressure subjects, cooperation decreases with date, but not among time delay subjects. As a result, the positive effect of time pressure is predicted to decay over time. 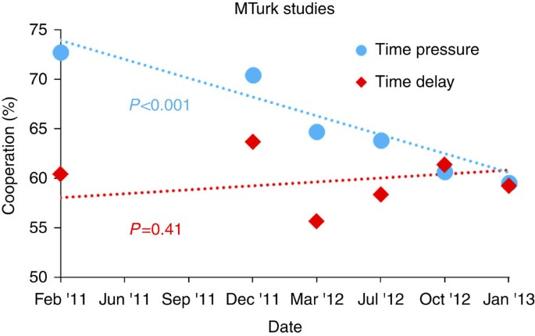Figure 3: The effect of time pressure on cooperation decayed as the MTurk subject pool became more experienced. Percentage of endowment contributed to the public good is shown, for subjects that obeyed the time constraint. For visualization periods, date is rounded down into 100-day bins. To make cooperation levels comparable across studies, only data from US residents is plotted, as there are different baseline average levels of cooperation across subject pools from different countries, and later studies restricted to the United States only. Note that the first bin includes RGN Study 6 as well as two other MTurk studies run shortly thereafter. Trend lines andP-values generated by linear regression with robust s.e. values clustered on IP address, not including controls. Regression results are shown in Table 3 , and the data are visualized in Fig. 3 . We focus on the regressions that include controls because certain important demographic factors varied systemically over time (in particular, many later studies excluded subjects living in India, who contribute less than American subjects on average; see Table 1 ). First we consider subjects who obeyed the time constraint (column 2; P -values generated using linear regression with robust s.e. values). As predicted, we find a significant negative interaction between time pressure and date (coefficient=0.0002, P <0.0001), as well as a significant positive coefficient for time pressure (coefficient=0.152, P <0.0001) and a non-significant coefficient for date (coefficient=0.00003, P =0.543). Evaluating the net coefficient (that is, the coefficient for date among subjects in the time pressure condition) shows a significant decrease in cooperation over time (coefficient=−0.0002, P <0.0001). When considering all subjects (column 4), the results are qualitatively equivalent, with all key findings statistically significant. Table 3 Regression results examining cooperation as a function of the interaction between time pressure and date among the 12 studies conducted on MTurk. Full size table Figure 3: The effect of time pressure on cooperation decayed as the MTurk subject pool became more experienced. Percentage of endowment contributed to the public good is shown, for subjects that obeyed the time constraint. For visualization periods, date is rounded down into 100-day bins. To make cooperation levels comparable across studies, only data from US residents is plotted, as there are different baseline average levels of cooperation across subject pools from different countries, and later studies restricted to the United States only. Note that the first bin includes RGN Study 6 as well as two other MTurk studies run shortly thereafter. Trend lines and P -values generated by linear regression with robust s.e. values clustered on IP address, not including controls. Full size image The significant coefficient on time pressure indicates that at the time of the initial RGN study, cooperation was significantly higher under time pressure than under time delay. The non-significant coefficient on date indicates that among subjects in the time delay condition, cooperation has not changed across time. Moreover, the significant negative interaction between time pressure and date (along with the significant net coefficient) indicates the cooperation of time-pressured subjects has decreased over time. (Critically, the initial RGN experiment is not the only study to get a large effect, as shown in Fig. 1 ; therefore this decrease in effect size is not simply a series of null results following the initial success of RGN, and the effect we are describing is not regression to the mean. Furthermore, Fig. 3 clearly shows a systematic decrease in cooperation under time pressure in the span of 2 years.) Thus, we demonstrate that the time pressure effect reported in RGN Study 6 has incrementally decayed over time, suggesting that increasing experience with economic games among MTurk subjects undermines cooperative intuitions. To provide additional evidence that this decay involves subjects becoming more experienced, we ask whether decision times themselves have decreased over this 2-year period. If so, this would suggest that subjects were becoming increasingly familiar with the cooperation tasks. 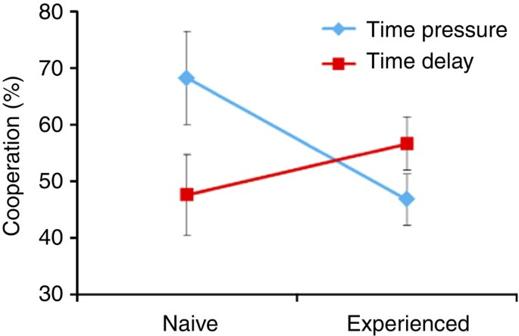Figure 4: Experience moderates the effect of time pressure in a PGG framed as resource extraction. Percentage of endowment not extracted from the common pool is shown on theyaxis, for subjects that obeyed the time constraint. Subjects under time pressure had to decide within 7 s. Subjects under time delay had to wait at least 10 s before deciding. Naïve subjects are those who reported no previous experience with similar MTurk studies in a post-experimental questionnaire. By assessing experience, this experiment replicates within one study the cross-study pattern observed inFig. 3. Error bars indicate s.e.m. Number of observations: pressure naïve, 25; delay naïve, 41; pressure experienced, 87; delay experienced, 93. Indeed, as shown in Table 4 , we find a significant correlation between decision time and date, in both conditions combined (linear regression with robust s.e. values; coefficient=−0.0002, P <0.001) and in the time pressure condition in particular (linear regression with robust s.e. values; coefficient=−0.0001, P <0.001), and also when including subjects who did not obey the time constraint (linear regression with robust s.e. values; both conditions: coefficient=−0.0001, P <0.001; time pressure only: coefficient=−0.0002, P <0.001). Table 4 Regression results examining log10-transformed decision time as a function of date among the 12 studies conducted on MTurk. Full size table Direct demonstration of experience moderating the effect of time pressure Finally, we directly link the decline in time pressure effect shown in Fig. 3 to experience. Building on the results of our aggregate analysis, we conducted a final additional experiment on MTurk in April 2013. We recruited 284 subjects living in the United States to participate in a one-shot PGG under time pressure or time delay. To reduce subjects’ level of familiarity with the decision setting, we altered the framing of the game to make it less obviously similar to previous PGGs: we framed the subjects’ decision as extracting tokens from a common pool, rather than contributing to a common project (all tokens left in the pool are doubled and split equally amongst four players). We also altered the number of tokens (2,000 per subject) and the exchange rate (100 tokens=1 cent). We did not, however, change the multiplier on cooperation (2 × ) or the number of players (4). Thus the strategic setting faced by the subjects is identical to the PGG used in RGN. We addressed the fact that decision times have been decreasing on MTurk by reducing the time limit in the time pressure condition to 7 s rather than 10 s (so as to more effectively apply pressure to subjects’ decision-making process). In the time delay condition, subjects were asked to wait 10 s before deciding, as in RGN. We also took this opportunity to demonstrate the robustness of the RGN findings by making several modifications to the experimental design. As in some of the later studies included in our aggregate analysis (but unlike RGN), we (i) included a timer that counted down in the time pressure condition, and counted up in the time delay condition (so that subjects would not have to keep track of elapsed time themselves), and (ii) changed the decision input to a set of radio buttons with no default selected (rather than a slider initialized to 50%, as in RGN). As a result of the timers, the fraction of subjects obeying the time constraint was much higher than in RGN (84% in time pressure, 92% in time delay). Finally, to demonstrate that time pressure effects are not driven by lack of comprehension, we included comprehension questions prior to the extraction decision (and prior to the application of time pressure or delay), rather than afterwards as in RGN. See Supplementary Methods for full experimental instructions. We assessed the role of experience in moderating time pressure by asking subjects ‘to what extent have you previously participated in other studies like to this one (that is, that involve the dividing up of money)?’ answered on a 5-point Likert scale with 1=nothing like this scenario, 3=something like this scenario and 5=exactly this scenario. Our analysis classifies subjects selecting 1 as ‘naïve,’ and subjects selecting 2 through 5 as ‘experienced.’ Experience was assessed at the end of the experiment as one of many demographic questions, rather than as a screening question at the beginning of the experiment. This minimizes the incentive for subjects to misreport their prior experience in order to be eligible for the study. Importantly, the fraction of naïve subjects did not differ significantly between the time pressure and time delay conditions (λ 2 test: only subjects that obeyed the time constraint, P =0.204; all subjects, P =0.121). This final experiment was designed to test the hypothesis that increasing subject pool experience is responsible for the decay in time pressure effect on MTurk demonstrated above. Thus we predict that this experiment will reproduce within a single study the cross-study patterns observed in Fig. 3 : (i) a significant interaction between time pressure and experience, such that (ii) time pressure will increase cooperation among naïve subjects but not experienced subjects, and (iii) experience will decrease cooperation among subjects under time pressure but not among subjects under time delay. The results are shown in Fig. 4 . Regressions are shown in Table 5 ( P -values generated using linear regression with robust standard errors, including controls for comprehension, age, gender, education, social and fiscal conservatism, and belief in God). As predicted, there is a highly significant interaction between time pressure and experience (column 2, coefficient=0.350, P =0.008). As a result, there is a significant positive effect of time pressure on cooperation among naïve subjects (as indicated by the time pressure dummy, coefficient=0.230, P =0.041), while evaluating the net coefficient for time pressure among experienced subjects shows a non-significant effect of time pressure trending in the opposite direction (coefficient=−0.119, P =0.072). Similarly, we find no significant effect of experience in the time delay condition (as indicated by the experience dummy, coefficient=0.093, P =0.295), while evaluating the net coefficient for experience among time-pressured subjects shows a significant negative effect of experience (coefficient=−0.256, P =0.008). Qualitatively equivalent results with all key findings statistically significant are obtained when including subjects that disobeyed the time constraint (column 4). We also note that similar results are achieved when interacting the time pressure dummy with log 10-transformed total number of academic studies completed, rather than the naïve versus experienced categorization used above (interaction term: coeff=−0.150, p=0.045 using only subjects that obeyed the time constraint; coefff=−0.149, p=0.027 using all subjects). Thus, we successfully reproduce the cross-study pattern from Fig. 3 within a single study using experience as a moderator of the time pressure effect, validating the prediction of the SHH. Figure 4: Experience moderates the effect of time pressure in a PGG framed as resource extraction. Percentage of endowment not extracted from the common pool is shown on the y axis, for subjects that obeyed the time constraint. Subjects under time pressure had to decide within 7 s. Subjects under time delay had to wait at least 10 s before deciding. Naïve subjects are those who reported no previous experience with similar MTurk studies in a post-experimental questionnaire. By assessing experience, this experiment replicates within one study the cross-study pattern observed in Fig. 3 . Error bars indicate s.e.m. Number of observations: pressure naïve, 25; delay naïve, 41; pressure experienced, 87; delay experienced, 93. Full size image Table 5 Regression results examining cooperation in the PGG extraction experiment. Full size table The present results illuminate the cognitive basis of cooperation. We introduced the SHH as a theory that explains why intuition tends to support cooperative decision making, and for whom intuition will favor selfishness. We then tested the predictions of the SHH by examining the effect of time pressure on cooperation in a set of cooperation experiments with monetary stakes. Combining all fifteen such experiments our lab ran over a 2-year period, we found strong evidence that on average time pressure increases cooperation relative to time delay (even when including subjects who failed to obey the time constraint). Thus we have demonstrated a causal relationship between time pressure and cooperation. We also found that there is substantial variation at the study level in the effect of time pressure on cooperation. From study to study, the effect of time pressure varies from large and positive to 0, but is never significantly negative. Finally, we provided an explanation for this variation: substantial previous experience with one-shot anonymous laboratory games undermines cooperative intuitions, by giving subjects a chance to remodel their automatic responses. Our results help to reconcile previous contradictory findings regarding time pressure and cooperation. The two time pressure studies reported in RGN found that time pressure increased cooperation relative to time delay [12] . A subsequent set of experiments, however, found no significant effect of time pressure on cooperation across five studies [17] . In four of these studies, the design differed from that of RGN in ways that could have undermined any time pressure effect [41] . Subjects completed a number of economic decisions unrelated to cooperation immediately prior to the cooperation games, potentially giving them an opportunity to adjust to the laboratory setting. They then made a series of cooperation decisions where the returns to cooperation were varied, with time pressure applied to each decision. Thus, the time pressure affected not only their decision-making process, but also their ability to understand the payoff structure. Finally, after learning the basic game structure, but before beginning the cooperation games, subjects were informed that time pressure would be applied to their subsequent decisions (unlike in RGN, where subjects were not informed about the time pressure/delay until immediately before they had to make their decision). This design choice seems likely to reduce the efficacy of the time constraint manipulation. The fifth study, however, used a similar design to RGN, yet also found no significant effect of time pressure (although we note that in the treatment closest to the design of RGN, there was a trend in the expected positive direction). The null results of this final study fit within the pattern revealed in Fig. 1 , where numerous studies also find null effects (despite an overall significant positive effect of time pressure). As the level of previous experience of subjects was not assessed in any of these previous studies, we cannot say whether experience was the key moderator explaining the difference from RGN, or whether some other factor (such as interpersonal trust) is primarily responsible the observed differences. Whatever the correct explanation is, the conceptual framework and results we present here emphasize the importance of considering potential individual difference moderators in future time pressure studies. Our theory and results are also consistent with research using other manipulations of intuitive versus reflective decision making, as well as research using games other than the PGG to study prosociality. For example, priming an intuitive versus reflective mindset by having subjects write about a time in their lives when intuitive decision making worked out well (or when reflective decision making worked out poorly) increased cooperation in the PGG on average, but not among experienced subjects [12] . Similarly, promoting intuitive judgment by having subjects perform a cognitively demanding task while making their decision (that is, applying ‘cognitive load’) increased fairness in a zero-sum resource allocation game [42] . Applying cognitive load to the Dictator Game, where subjects unilaterally decide how much money to give to an anonymous stranger, was found to increase giving in one study [43] , to have no effect in a second study [44] , and in a third study to increase giving for some subjects but not others, depending on the perceived interpersonal closeness of the interaction partner [45] . It has also been found that impairing the function of the right lateral prefrontal cortex, a brain region associated with deliberation and control, increases giving in a unilateral money transfer, while amplifying this region decreases giving [46] ; that individuals with little self-control are more likely to make sacrifices for the benefit of their romantic partners [47] ; that people by default project a cooperative frame onto neutrally framed prisoner’s dilemma games [48] ; and that young children often spontaneously help others [49] , [50] . These results further reinforce our conclusion that intuitive processes promote prosociality for some people, and have no effect for others, but do not systematically decrease prosociality. This pattern of study-level variation is consistent with the predictions of the SHH, and indicates the existence of moderators of the effect of intuition. We provide evidence for one such moderator predicted by the SHH, the experience of the subject pool: the size of the time pressure effect on MTurk decreased significantly over a 2-year period as MTurk workers have become increasingly experienced. We directly demonstrate the moderating effect of experience on time pressure in a final experiment where experience was assessed in a post-experimental questionnaire. Time pressure increased cooperation among naïve but not experienced subjects. While providing further evidence for the SHH, the decay of the time pressure effect on MTurk poses practical challenges. MTurk is an extremely powerful, and popular, experimental platform. Yet our results suggest that certain types of studies may be difficult to run on MTurk due to the extremely high level of experience we demonstrate among MTurk subjects. When using lab experiments meant to expose the misapplication of intuitions developed in daily life, it is important to have a largely naïve subject pool. Alternatively, one may seek to employ novel paradigms with which subjects will have had less experience. This raises an important topic of future research: to what extent can individuals generalize experiences or decisions across different economic games and across different decision settings more broadly? Our final study further demonstrates the robustness of the time pressure effect to variation in experimental design details: First, the cooperation decision was framed as choosing not to extract from a common pool rather than choosing to contribute to a common project. Second, timers indicating the elapsed time were provided. Third, decisions were input using radio buttons rather than a slider with a default response. Finally, comprehension questions were asked before the decision rather than afterward. Nonetheless, time pressure significantly increased cooperation among naïve subjects. Furthermore, the intuitive cooperation effect cannot be explained by time pressure causing subjects to make more errors and thus behave more randomly. If this were true, average contributions in the conditions increasing intuitive processing (pro-intuition primes and time pressure) would be closer to 50% than contributions in more reflective conditions (pro-reflection and time delay). This is not, however, what we observe in Fig. 4 . The same is true of RGN, where the average reflective contribution was closer to 50% than the average intuitive contribution in all studies. We note that in our final study, we assessed experience using a self-report Likert scale. Such a measure is not ideal, as it is open to misrepresentation by subjects who misremember their previous experience or who purposefully lie. (Subjects may lie because they think their answer will affect eligibility to participate in future studies). Developing non-self-report measures to screen out highly experienced MTurk workers is an important direction for future work using MTurk. Furthermore, experience is not the only factor likely to moderate subjects’ intuitive responses. For example, the SHH predicts that cultural and institutional factors (effecting whether cooperation is advantageous or disadvantageous in daily life) will also effect whether cooperation is intuitive. Thus we would not expect time pressure to always increase cooperation, even among naïve subjects. Further identification of specific factors that moderate the effect of time pressure, and intuition more generally, on cooperation is an important direction for future research. The SHH connects to economic models of social preferences. Past experience can directly influence current behaviour in one-shot anonymous games if subjects have preferences that incorporate beliefs about how others will behave [51] , [52] , [53] , [54] , [55] , [56] , [57] , [58] : interacting with largely cooperative partners in daily life may lead to an increased expectation that partners will cooperate in the lab. Upon reflection, however, people may realize that this is an overgeneralization, as the structures that make cooperation advantageous in daily life are absent in the lab. Past experience can also affect behaviour by directly remodelling preferences, for example by increasing the disutility that subjects intuitively experience from unequal outcomes [59] , or the utility experienced from efficient outcomes [60] . Subjects may, upon reflection, counter these intuitive preferences and reduce their weighting in the utility function. Experimental evidence that previous experience changes subsequent giving in the Dictator Game, particularly among subjects who rely on heuristics, is suggestive of true remodelling of preferences [25] . Further distinguishing the extent to which the SHH operates via beliefs versus preferences in an important direction for future research. The SHH also connects to theories of ‘generalized reciprocity’ or paying-it-forward, in which others cooperating with oneself induces one to cooperate more readily with third parties in the future [61] , [62] , [63] , [64] . Unlike direct and indirect reciprocity, upstream reciprocity is not in general a mechanism for the evolution of cooperation [62] . Thus, the SHH predicts that reflection should undermine such behaviour. Moreover, the SHH sheds light on behaviour in settings where identifying the self-interested strategy is cognitively demanding. The SHH predicts that the more challenging is to determine the optimal behaviour in the current setting, the greater the role of intuition will be (as reflection is impaired by not ‘knowing the right answer’). Thus in demanding tasks—for example, fixed-length cooperation games that require backward induction to solve [65] , [66] , [67] —people’s behaviour should more faithfully reflect the strategies that are advantageous for them in daily life. For most of the American undergraduates typically participating in such experiments, the default is likely to be cooperation. The SHH therefore helps to explain why experiments often observe substantial cooperation in finite length games, and why more cooperation is observed in longer games (where more induction is required to reach the non-cooperative solution) [67] . Further evidence in support of this interpretation comes from the observation that slower responses in fixed-length games tend to begin defecting earlier on in the game, suggesting a greater degree of backward induction [68] . Examining the SHH through the lens of evolutionary dynamics is an important direction for future research: could natural selection lead to the evolution and maintenance of such a learning strategy? There is good reason to expect that the answer will be yes. Deliberation may be costly, relative to a heuristic response, if the heuristic response leads to advantageous behaviour most of the time and if the deliberation process is error prone. Likewise, automated social behaviour may be advantageous because it is quicker or because it signals a stable disposition to potential interaction partners. Thus, it may be advantageous to rely on social heuristics that are well tuned to the environment, producing behaviours that perform well on average. Furthermore, individual learning may play a critical role in this tuning process if social environments are variable across populations (making genetically programmed behaviour undesirable), but fairly stable within any given individual’s environment (making learned behaviours generalizable). These on-average optimal responses will, however, be sub-optimal in some subset of cases, and over time, the response that is on-average optimal is likely to change. Thus, it may sometimes be worth paying the cost of reflection. Evolutionary game theoretic models of dual-process agents may extend this line of thinking, yielding a formal theory of the conditions under which natural selection favors agents that combine intuition and deliberation. In sum, our results provide evidence that social intuitions acquired in daily life spill over into one-shot anonymous interactions. These intuitions, however, may be countered by experience with, or explicit knowledge of, the atypical conditions that prevail in the laboratory. This dual-process framework successfully organizes a large amount of data concerning the relationship between intuition and cooperation and provides a foundation for future research on the cognitive basis of prosocial behaviour. Data used in aggregated analyses We analyse data from 15 different time constraint studies, resulting in 6,913 decisions by 5,832 unique individuals. To avoid ‘file-drawer effects’ and other biases through which negative or contradictory results can be suppressed [69] , [70] , we analyse all data applying time pressure or delay to cooperation that we collected between February 2011 and February 2013: we include all studies in which subjects (i) were randomized into either time pressure or time delay while (ii) deciding whether to pay a cost to give a greater benefit to one or more others. This includes the data published in 2012 by RGN [12] (the first two such experiments we ran) as well as data from studies we are currently preparing for publication, as well as failed pilots, abandoned projects, experimental designs we subsequently reconsidered, and so on. While each of these studies varies in its details, they all involve the application of time pressure/delay to cooperation decisions. All studies were approved by the Committee on the Use of Human Subjects at Harvard University and involved no deception. We now provide information regarding the elements that varied across studies (also summarized in Table 6 ). Table 6 Description of each study included in our aggregate analysis. Full size table Recruitment: twelve studies were conducted using MTurk [35] , [36] , [37] , [38] , [39] , [40] (nine of these were restricted to residents of the United States); one study was conducted using the international online subject pool maintained by Yale University (eLab); and two studies were conducted in the (physical) Harvard Decisions Sciences Laboratory at the Harvard Kennedy School. Cooperation measure: Nine studies measured fraction contributed in a single one-shot four-person linear PGG with a 2 × contribution multiplier; one study measured fraction contributed in a series of 15 one-shot (stranger matching) four-person linear PGGs with a 2 × contribution multiplier (subjects were told the outcome of each PGG before proceeding to the next); two studies measured fraction sent to partner in a single one-shot continuous Prisoner’s Dilemma (PD) with a benefit-to-cost ratio of 2; one study measured probability of cooperating in a single one-shot binary PD with a benefit-to-cost ratio of 7/3; 1 study measured amount sent by Player 1 in a single one-shot trust game where Player 1 transfers were tripled; and 1 study measured amount transferred in a hypothetical (unincentivized) Dictator Game where transfers where doubled. Comprehension checks: In each of these studies, after making their decisions, subjects were asked two comprehension questions to assess their understanding of the social dilemma they faced: what decision maximizes the group’s earnings, and what decision maximizes the individual’s earnings. The only exceptions are as follows. In the binary PD and the trust game, subjects were asked to do two payoff calculations rather than the qualitative questions; in one of the 1-shot PGG experiments, half of the subjects answered the comprehension questions before making their decision rather than after; and in the 15-round stranger-matching PGG, instructions were read aloud in the lab, questions were answered and comprehension was confirmed orally prior to the beginning of the session. Time pressure/delay manipulation: In all studies, subjects under time pressure were asked to respond as quickly as possible and told they had at most 10 s (with one exception, see below), while subjects under time delay were asked to carefully consider their decision before responding and told to wait at least 10 s before answering. In eight studies, subjects were then allowed to enter their decision at any time. In four studies, a timer counted down from 10 s in time pressure and a timer counted up from 0 s in time delay, and subjects were allowed to enter their decision at any time. In two studies, a timer counted down from 10 s in time pressure and subjects were allowed to enter their decision at any time; and a timer counted up from 0 s in time delay, and subjects were randomized into settings where they either (i) could answer at will, (ii) could select an answer at will but were forced to wait at least 10 s before submitting their decision, or (iii) had to wait 10 s before being allowed to make any selection. In one study (the 15-round stranger matching study), subjects in time pressure were given only 8 s to respond, a timer counted down from 8 s, and subjects who did not respond in time were assigned a random contribution amount, enabling the game to continue (this occurred in only 2.6% of time pressure decisions, and subjects were informed of this ahead of time; these random contribution decisions are of course excluded from our analysis); in time delay, subjects were forced to wait 10 s before being allowed to enter a contribution amount. Secondary manipulations: In eight of these studies, time pressure versus delay was the only experimental manipulation. In the other seven studies, time pressure versus delay was crossed with another manipulation (for example, an alternative framing of the game, specific information about the other players, alternative order of comprehension questions, and so on); in our analyses, we aggregate across secondary manipulations. Demographics: In all studies, subjects completed a questionnaire after making their decision. Although the contents of the questionnaire varied across studies, basic demographic information was collected in all studies (age, gender, education level, country of residence). Missing demographic data are interpolated at the study level: Subjects for whom age, gender or US residency information is missing are assigned the mean value for their study, and subjects for whom education level information is missing are assigned to the ‘Unknown’ category. Statistical methods All analysis is conducted using linear regression taking normalized cooperation amount (0=maximum selfishness, 1=maximum cooperation) as the dependent variable. To account for the non-independence of multiple observations from the same subject, we use robust s.e. values clustered on subject. For online studies, we use IP address as the subject identifier (that is, we treat multiple decisions from the same IP address as coming from the same subject). All regressions include a binary (‘dummy’) variable indicating decision making under time pressure. All regressions control for study-level variation in cooperate rates by including dummy variables for each of the 15 studies, taking RGN Study 6 (‘Study A’) as the (arbitrary) baseline. When controlling for education, we take ‘less than a high school degree’ as the baseline and include dummies for ‘high school diploma’, ‘vocational training’, ‘attended college’, ‘bachelor’s degree’, ‘graduate degree’, and ‘unknown’. When controlling for country of residence, we take the United States as the baseline and include a dummy for residing in India and a dummy for residing in any country other than the United States or India (as most MTurk workers are either from the United States or India). How to cite this article: Rand, D. G. et al. Social heuristics shape intuitive cooperation. Nat. Commun. 5:3677 doi: 10.1038/ncomms4677 (2014).